Symbiotic adaptations in the fungal cultivar of leaf-cutting ants Centuries of artificial selection have dramatically improved the yield of human agriculture; however, strong directional selection also occurs in natural symbiotic interactions. Fungus-growing attine ants cultivate basidiomycete fungi for food. One cultivar lineage has evolved inflated hyphal tips (gongylidia) that grow in bundles called staphylae, to specifically feed the ants. Here we show extensive regulation and molecular signals of adaptive evolution in gene trancripts associated with gongylidia biosynthesis, morphogenesis and enzymatic plant cell wall degradation in the leaf-cutting ant cultivar Leucoagaricus gongylophorus . Comparative analysis of staphylae growth morphology and transcriptome-wide expressional and nucleotide divergence indicate that gongylidia provide leaf-cutting ants with essential amino acids and plant-degrading enzymes, and that they may have done so for 20–25 million years without much evolutionary change. These molecular traits and signatures of selection imply that staphylae are highly advanced coevolutionary organs that play pivotal roles in the mutualism between leaf-cutting ants and their fungal cultivars. Obligate interspecific mutualisms have often produced synergistic co-adaptations that allowed them to use previously inaccessible resources [1] , [2] . To evolve higher levels of cooperative integration, such mutualistic co-dependencies need to remain bilaterally stable over long time spans, a restrictive condition that is far from always fulfilled [3] , [4] . When it is fulfilled, specialized morphological, behavioural and metabolic traits may evolve and ultimately lead to gene loss when interacting partners provide complementary functions [5] . Interspecific mutualisms may also represent different levels of integration. Many symbioses can be defined as ectosymbioses where partners have retained independent sexual reproduction in a fairly symmetrical way as, for example, many lichens, specialized pollination interactions and some mycorrhizal-plant symbioses [2] , [5] . Others are endosymbioses and have almost, per definition, asymmetrical reproduction, with one partner being dependent on the other. Here, symbionts are normally microorganisms or asexual fungi providing specific nutritional services in exchange for a predictable supply of limiting resources by multicellular animal or plant hosts [6] . Mutualistic symbioses that involve colonies of eusocial insects often have intermediate levels of integration, because interactions concern both the individual level and the colony level [7] . The clearest examples of this ambiguity occur in the ants and termites that convergently evolved fungus farming [8] , [9] . These symbioses rely on specialized ecto-interactions between individual workers and fungal tissues, while the entire clonal fungus garden functions as a protected endosymbiont of the colony [10] . In both farming systems, the crop fungi have evolved symbiotic organs: nodules in the Termitomyces termite cultivars as food packages that vector asexual spores to the faeces for intracolony symbiont propagation [8] and somatic staphylae with gongylidia in the fungus-growing ant cultivars to feed the ants while vectoring fungal enzymes to the faecal droplets used to enhance new fungal growth ( Fig. 1a,b ) [9] . 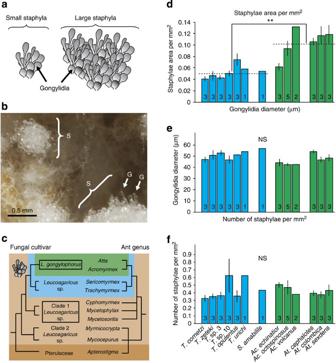Figure 1: Variation in gongylidia morphology amongTrachymyrmex,Sericomyrmex,AcromyrmexandAttafungus-growing ants. (a) Drawing of gongylidia and representative staphylae of different size. (b) Image of gongylidia (G) and staphylae (S) in the fungus garden of the leaf-cutting antA. echinatior. (c) Phylogenetic reconstruction of the coevolution of ant symbiotic fungi (left) and fungus-growing ant genera (right) based on previously published work9,11,12,23, with the origin of gongylidia marked. Boxed genera highlight the phylogenetic position of theA. echinatiorandC. longiscapusfungal cultivars used in the codon-based transcriptome comparison of the present study. Green: leaf-cutting ants cultivatingL. gongylophorus, blue: higher attine ants cultivating a variety ofLeucoagaricusspp. with gongylidia, light brown: lower-attine ants cultivating a diverse group of fungi without gongylidia from two clades (clade 1 and 2) in the family, Agaricaceae and Pterulaceae, cultivated by a subclade of ants in the genusApterostigma. (d) Mean total area (mm2) covered by staphylae (±s.e.) per mm2of fungus garden surface showing significantly higher cover proportions inAttaand (partially)Acromyrmexleaf-cutting ants (green) compared withTrachymyrmexandSericomyrmexhigher-attine ants (blue) (Kruskal–Wallis,H=27.4, df=12,P=0.007 **, mean values illustrated by horizontal dotted lines). (e) Gongylidia diameter (μm)±s.e. per fungus garden (Kruskal–Wallis,H=19.2, df=12, NS: Not Significant) and (f) Number of staphylae per mm2fungus garden (Kruskal–Wallis,H=10.7, df=12, NS: Not Significant). The number of sampled colonies per species is given inside each column. Figure 1: Variation in gongylidia morphology among Trachymyrmex , Sericomyrmex , Acromyrmex and Atta fungus-growing ants. ( a ) Drawing of gongylidia and representative staphylae of different size. ( b ) Image of gongylidia (G) and staphylae (S) in the fungus garden of the leaf-cutting ant A. echinatior . ( c ) Phylogenetic reconstruction of the coevolution of ant symbiotic fungi (left) and fungus-growing ant genera (right) based on previously published work [9] , [11] , [12] , [23] , with the origin of gongylidia marked. Boxed genera highlight the phylogenetic position of the A. echinatior and C. longiscapus fungal cultivars used in the codon-based transcriptome comparison of the present study. Green: leaf-cutting ants cultivating L. gongylophorus , blue: higher attine ants cultivating a variety of Leucoagaricus spp. with gongylidia, light brown: lower-attine ants cultivating a diverse group of fungi without gongylidia from two clades (clade 1 and 2) in the family, Agaricaceae and Pterulaceae, cultivated by a subclade of ants in the genus Apterostigma . ( d ) Mean total area (mm 2 ) covered by staphylae (±s.e.) per mm 2 of fungus garden surface showing significantly higher cover proportions in Atta and (partially) Acromyrmex leaf-cutting ants (green) compared with Trachymyrmex and Sericomyrmex higher-attine ants (blue) (Kruskal–Wallis, H =27.4, df=12, P =0.007 **, mean values illustrated by horizontal dotted lines). ( e ) Gongylidia diameter (μm)±s.e. per fungus garden (Kruskal–Wallis, H =19.2, df=12, NS: Not Significant) and ( f ) Number of staphylae per mm 2 fungus garden (Kruskal–Wallis, H =10.7, df=12, NS: Not Significant). The number of sampled colonies per species is given inside each column. Full size image The gongylidia of attine ant cultivars offer unique opportunities for unravelling the molecular mechanisms of fungal co-adaptation to domesticated life. The obligate dependence of the attine ant tribe to farming fungi for food goes back ca . 50 million years. This evolutionary innovation allowed the single ancestor of the attine ants to become a functional decomposer [9] , but the crop fungi that are reared by extant basal attine genera did not become reproductively isolated from free-living relatives for the first 25–30 million years [11] . Obligate crop status finally evolved 20–25 million years ago (MYA) with the emergence of the gongylidia-bearing staphylae, a transition that initiated diversification into four evolutionarily derived genera of ‘higher’ attine ants ( Trachymyrmex , Sericomyrmex , Acromyrmex and Atta ), all of which rear descendants of this first gongylidia-bearing symbiont ( Fig. 1c ) [11] , [12] . Relative to fungal hyphae, the gongylidia have high concentrations of lipids and carbohydrates (free sugars and polysaccharides) and provide all food for the ant larvae and most food for the adult ants [13] . Based on comparisons of extant species, the evolution of gongylidia coincided with distinct changes in fungus garden enzyme activity [14] , proportional shifts in plant material used as fungal substrate [15] and the cultivated fungi loosing the ability to live independently without the ants [10] . One of the most striking co-evolutionary adaptations is that the ants do not digest many of the fungal enzymes they ingest when consuming gongylidia, but deposit them with the faecal fluid on chewed-up plant material that they incorporate at the top edges of their gardens [16] , [17] . This implies that the stationary fungus garden uses the ants to vector fungal enzymes from the most productive central garden sections to peripheral top layers where new substrate is abundant but mycelial growth is sparse [18] . Faecal droplet protein analysis by mass spectrometry has so far identified 33 partial amino acid sequences in faecal fluid of the leaf-cutting ant Acromyrmex echinatior [19] . At least 14 of these are enzymes and now documented to be produced by the L. gongylophorus cultivar (Agaricaceae: Basidiomycota) [16] , including seven cell-wall-degrading pectinases, six proteinases and a laccase enzyme that detoxifies plant defensive phenolic compounds [19] , [20] , [21] . Except for a single pectinase and protease, all of the genes coding for these enzymes were overexpressed in the gongylidia, suggesting that the enzymes have been under selection to remain active after passing through the ant guts, a scenario that is supported by molecular evidence for positive selection of specific amino acids in the laccase gene [20] . The considerable metabolic investment in mass production of staphylae with gongylidia ( Fig. 1b ) thus appears to represent a major co-adaptation characterizing the transition to higher attine fungus farming [10] , [22] . In the present study, we aimed to quantify the extent to which co-evolutionary selection has shaped the morphology of gongylidia and modified their molecular functionality to first resolve key phenotypic questions of their functional significance before embarking on a molecular analysis of the genetic underpinning of such functions. In particular, we asked whether: (I) the origin of gongylidia as a key innovation among ant fungal cultivars 20–25 MYA [11] was followed by significant secondary morphological modification in specific genera of farming ants, (II) the fundamental phenotypic modifications of hyphal-tip growth that produced the gongylidia are related to genomic changes in nucleotide composition or differential gene expression relative to ‘lower’ attine ant cultivars that do not produce gongylidia, (III) nutritional complementarity has selected for essential amino acids that the ants are unable to produce, being offered by the fungal gongylidia and (IV) the expression of carbohydrate-active fungal enzymes is upregulated in gongylidia, similar to what has been shown for pectinases [19] , proteinases [21] and a laccase enzyme [20] . To answer these questions, we first measure the morphological diversity of gongylidia in natural field-collected fungus gardens of six species of Atta and Acromyrmex leaf-cutting ants and seven species of Trachymyrmex and Sericomyrmex higher-attine non-leaf-cutting ants. After establishing that staphylae size in leaf-cutting ant fungi has increased over evolutionary time, but that the morphology of individual gongylidia appeared to be conserved, we then proceed with RNA-sequencing to obtain genome-wide transcriptomes. This allows us to compare gongylidia-specific and undifferentiated mycelium transcriptomes of L. gongylophorus reared in three A. echinatior laboratory colonies, to determine the extent to which gongylidia prioritize producing amino acids and carbohydrate-active enzymes that the ants need for their functions in the mutualism. Third, we estimate rates of non-synonymous and synonymous base changes (dN/dS) in the L. gongylophorus symbiont of A. echinatior from comparisons with homologous genes in lower attine ant cultivars that do not produce gongylidia. We therefore also acquire mycelial transcriptomes of two Leucoagaricus sp. cultivars of Cyphomyrmex longiscapus ( Fig. 1c ) that belong to the large and diverse sister clade (clade 1) of the cultivars that produce gongylidia [9] , [11] , [23] . Our analyses show extensive regulation and molecular signals of positive selection in gene trancripts associated with gongylidia morphogenesis and enzymatic plant cell wall degradation in the leaf-cutting ant cultivar L. gongylophorus. The fungus produces amino acids that the ants lack even though they are probably essential for ant development. Our results are consistent with a high degree of co-evolutionary integration in the higher attine fungus-growing ants. Gongylidia growth characteristics Morphological measurements of gongylidia in field-collected fungus gardens showed that staphylae (clusters of gongylidia; Fig. 1a ) covered a significantly larger area in leaf-cutting ant gardens than in gardens of higher-attine non-leaf-cutting ants (Kruskal–Wallis, H =27.4, df=12, P =0.007, Fig. 1d ). However, individual gongylidia size (mean diameter±s.e.=48.1±0.96 μm, Kruskal–Wallis, H =19.2, df=12, P =0.085, Fig. 1e ) and the number of staphylae per mm 2 of garden surface area (mean±s.e.=0.4±0.03, Kruskal–Wallis, H =10.7, df=12, P =0.553, Fig. 1f ) did not differ between fungus gardens cultivated by these two groups of farming ants. This implies that the mean size of the staphila organ has changed over evolutionary time, but not its overall number or the mean size of its gongylidia components. Coefficients of variation (CV) in leaf-cutting ant gardens were largest for the number of staphylae per mm 2 (mean CV±s.e.=25.3±5.6) and proportional staphylae cover per mm 2 (22.2±4.0) and lowest for gongylidia size (9.4±1.3), and these differences were even more pronounced for Trachymyrmex and Sericomyrmex cultivars (mean CV±s.e. number of staphylae per mm 2 =33.0±7.7; area covered by staphylae per mm 2 =21.7±2.9; gongylidia size=9.3±2.1). This shows that variation in gongylidia diameter and staphylae coverage have remained essentially unchanged, but that the number of staphylae per unit of garden surface became less variable in the leaf-cutting ant cultivar L. gongylophorus . The leaf-cutting ant symbiont surface thus appears as a dense uniform cover of staphylae of similar size, whereas gardens of Trachymyrmex and Sericomyrmex offer a lower and less uniform gongylidia harvest to the farming ants. Gongylidia diameter remained remarkably constant, both in overall mean and in spatial and evolutionary variation, indicating that transcriptomic comparisons are unlikely to be confounded by uncontrolled size variation of gongylidia. Transcriptome sequence annotation RNA-derived complementary DNA libraries from both gongylidia and mycelium of L. gongylophorus cultivated by A. echinatior were obtained from three colonies ( Ae322 , Ae331 and Ae376 ) using a combination of Illumina Hiseq2000 and 454-FLX Titanium sequencing ( Table 1 and Supplementary Table 1 ). All sequences from a single colony ( Ae322 ) were assembled into a reference transcriptome consisting of 23,110 contigs with a mean transcript size of 1,346 bp and an N50 of 1,950 bp ( Table 1 ), which is within the range (1.134–1.840 bp) of the average coding sequence length observed in other Basidiomycota, indicating that the assembly contained many full-length transcripts [24] . Blastx searches against the UniProtKB database yielded 17,621 (76%) transcripts with a significant hit ( e -value=10 −6 , Table 1 ), which corresponded to 9,107 unique accession numbers. Moreover, these were within the numerical range (6.522–20.614) of predicted coding genes in other Basidiomycota, indicating that our extraction and sequencing procedures covered most of the L. gongylophorus transcriptome. The number of significant hits was lower than the total number of hits, because functional polyploidy of the fungal cultivar [25] implies that multiple allelic transcript variants with similarly significant hits are expressed in each cultivar sample. Table 1 Summay of L. gongylophorus transcriptome assembly. Full size table Most transcripts mapped to the genomic sequence database of a L. gongylophorus strain from another A. echinatior colony (90%, 20,807/23,110, NCBI accession code PRJNA62733) [20] and an L. gongylophorus strain from an Atta cephalotes colony (90%, 20,690/23,110, NCBI accession code PRJNA48091) [26] , both from the same location in Panama, confirming that our laboratory procedures primarily extracted material form L. gongylophorus , and that symbiont strains reared by sympatric Acromyrmex colonies are very similar, consistent with earlier findings [27] . Of the 17,621 transcripts with a positive hit in the UniProtKB database, 99% (17,384) mapped to the Ascomycota and Basidiomycota ( Table 1 ), but we retained all 23,110 transcripts to avoid missing potentially novel transcripts not covered in the incomplete (7–15 × coverage) draft genome assemblies that were available. A total of 4,905 (21%) of the transcripts did not have either a UniProtKB, NCBI or Pfam hit, and were therefore regarded as orphans, whereas 11,867 (51%), 11,992 (51%) and 12,037 (51%) transcripts could be assigned a Pfam domain, be assessed for Gene Ontology, or be classified in EuKaryotic Orthologous Groups (KOG), respectively ( Table 1 ). Comparison of the L. gongylophorus transcriptome with three sequenced Agaricales genomes using bidirectional best blast hits yielded 4,927, 4,867 and 4,497 orthologous transcripts to Agaricus bisporus , Coprinopsis cinerea and Laccaria bicolor , respectively. Gene expression in gongylidia Patterns of genome-wide gene expression for gongylidia and mycelium across the L. gongylophorus cultivars of three A. echinatior colonies showed that 1,076 transcripts were significantly upregulated and 535 transcripts were significantly downregulated in gongylidia (log 2 fold-change >1.0, Benjamini–Hochberg adjusted P< 0.001, Fig. 2a and Supplementary Fig. 1 ). Many (43%; 697/1,611) of these differentially expressed transcripts could be assigned to a KOG group ( Supplementary Fig. 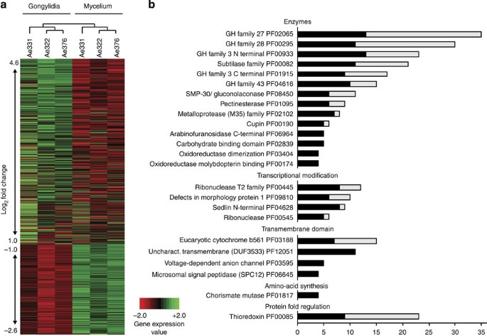Figure 2: Differentially expressed fungal genes between gongylidia and mycelium in threeA. echinatiorleaf-cutting ant laboratory fungus gardens. (a) Heat map showing biological variation in relative expression of the 1,076 significantly overexpressed (log2fold-change>1,P<0.0001) and the 535 significantly under-expressed (log2fold-change<−1,P<0.0001) transcripts. Relative expression values are scaled per transcript (row). (b) Pfam domains that were both highly expressed and significantly enriched (Bonferroni-adjustedP<0.05) in gongylidia relative to the total set of transcripts when using the hypergeometric distribution. Bars represent the number of Pfam domains in gongylidia (black) relative to the total number of Pfam domains present in both gongylidia and mycelium of theL. gongylophorustranscriptome (grey). Bars without a grey section thus represent domains for which all instances were among the highly expressed gongylidia transcripts. 2 ), and enrichment analysis of these KOG annotations showed that they were particularly involved in amino acid transport and metabolism (group E, Supplementary Table 2 ), intracellular trafficking, secretion, vesicular transport (group U, Supplementary Table 2 ) and inorganic ion transport and metabolism (group P, Supplementary Table 2 ). 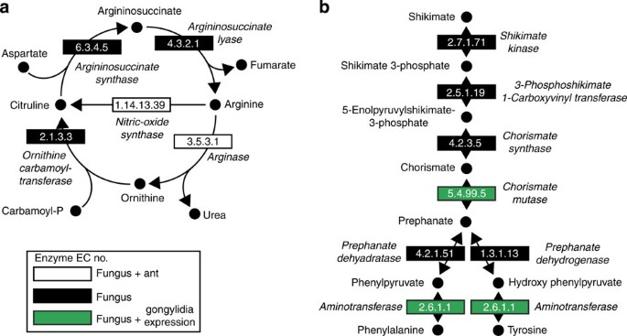Figure 3: Fungal symbiont genes coding for enzymes involved in the arginine and phenylalanine synthesis pathways. (a) The host antA. echinatiorhas lost the two enzymes argininosuccinate synthase (EC 6.3.4.5) and argininosuccinate lyase (EC 4.3.2.1)33, but the present transcriptome analysis shows that theL. gongylophorussymbiont possesses all the necessary enzymes for arginine synthesis (Supplementary Table 7). Ornithine carbamoyl-transferase (EC 2.1.3.3) was not found among any of the five Hymenopteran insects (A. cephalotes,Camponotus floridanus,Harpegnathus saltator,Apis mellifera,Nasonia vitripennis) that were previously analysed34, but was also identified in theL. gongylophorustranscriptome. (b) Two genes coding for enzymes mediating aromatic amino acids biosynthesis, chorismate mutase (EC 5.4.99.5) and aminotransferase (EC 2.6.1.1), had alleles that were significantly upregulated in the gongylidia (Supplementary Table 8), indicating that the essential amino acids phenylalanine and tyrosine are produced in high amounts in the gongylidia. The 25 transcripts with the highest read counts in gongylidia relative to mycelium included both carbohydrate-active pectinases and phenol-oxidizing laccases ( Supplementary Table 3 ). Figure 2: Differentially expressed fungal genes between gongylidia and mycelium in three A. echinatior leaf-cutting ant laboratory fungus gardens. ( a ) Heat map showing biological variation in relative expression of the 1,076 significantly overexpressed (log 2 fold-change>1, P< 0.0001) and the 535 significantly under-expressed (log 2 fold-change<−1, P< 0.0001) transcripts. Relative expression values are scaled per transcript (row). ( b ) Pfam domains that were both highly expressed and significantly enriched (Bonferroni-adjusted P< 0.05) in gongylidia relative to the total set of transcripts when using the hypergeometric distribution. Bars represent the number of Pfam domains in gongylidia (black) relative to the total number of Pfam domains present in both gongylidia and mycelium of the L. gongylophorus transcriptome (grey). Bars without a grey section thus represent domains for which all instances were among the highly expressed gongylidia transcripts. Full size image Using the hypergeometric distribution, further analysis of the 51% (547/1,076) upregulated genes that could be assigned to a Pfam domain revealed a significant overrepresentation of glycosyl hydrolase domains involved in carbohydrate degradation and of several regulatory protease, oxidoreductase and transmembrane domains ( Fig. 2b and Supplementary Table 4 ). In particular, the Pfam domain PF09810 that includes proteins affecting cellular morphology and mutation in the homologous YBR163w gene in Saccharomyces cerevisiae was overrepresented among the upregulated gongylidia transcripts ( Fig. 2b ). Active proteins with this domain often lead to slow growth and aberrant morphology with fragmented nuclei and mitochondrial defects [28] , consistent with gongylidia being growth-arrested somatic organs that will not have further cell division. Putative genes with signatures of positive selection Of the 35,901,080 available Illumina reads from the two sequenced C. longiscapus cultivars ( rmma110512-01 and jl130511- 03), 11,336,923 (70.7%) and 14,756,705 (74.3%) could be mapped to the L. gongylophorus reference transcriptome ( Supplementary Table 1 ). Subsequent phylogenetic analysis revealed nearly identical large subunit ribosomal RNA nuclear sequences, clustering together on the same clade 1 branch with Apterostigma auriculatum (accession code AF079592) and C. longiscapus S50 (accession code AF079597) when combined with published sequences [23] ( Supplementary Fig. 3 ). We therefore pooled the two C. longiscapus cultivar sequences to obtain better coverage, which resulted in 19,389 transcripts with mapped C. longiscapus cultivar reads. Orthology was inferred with bidirectional best blast hits resulting in 24.7% (5,708/23,110) transcript alignment pairs with an open reading frame (ORF) longer than 300 bp and thus amenable for further analysis. Pairwise calculation of the estimated ratio of non-synonymous to synonymous substitutions per site (dN/dS) showed an overall dN/dS ratio of 0.17 between L. gongylophorus and the C. longiscapus cultivar, confirming that most predicted ORFs evolve under strong purifying selection. Upregulated transcripts had a mean dN/dS ratio of 0.21, which was significantly higher than non-regulated transcripts (Welch’s t -test: t =2.03, df=235.4, P =0.0432). The mean dN/dS ratio of 0.18 among downregulated transcripts was not significantly different from non-regulated transcripts (Welch’s t -test: t =0.65, df=243.5, P =0.5188), indicating that elevated dN/dS ratios correlate with gene expression in gongylidia. Six transcripts had a dN/dS ratio>1, indicating positive selection for evolutionary modification at the nucleotide level ( Supplementary Table 5 ), but none of the non-synonymous changes were located in conserved transcript domains. Focusing on transcripts that were significantly upregulated in gongylidia and had a less-conservative cut-off ratio of dN/dS>0.5 provided eight transcripts (including three mentioned above, with dN/dS>1, Supplementary Table 6 ). Among these differentially regulated and structurally modified transcripts were sequences that encodes an extracellular metalloprotease, a regulatory protein kinase, a transcription factor and three transcripts that had sequence homology to uncharacterized basidiomycete proteins without Pfam domains that could indicate a potential function ( Supplementary Table 6 ). The most highly upregulated transcript of these uncharacterized sequences (contig18572, 506 bp) had a log 2 fold-change of 2.68 and also the highest observed dN/dS ratio of 3.587 ( Supplementary Table 6 ), but was an orphan with no sequence homology in the UniProt or Pfam databases. To identify putative function in intracellular pathways, the identified transcription factor and protein kinase were both searched with blastx against the Saccharomyces Genome Database [29] . This showed that the contig14212 transcript was homologous to the serine/threonine protein kinase Cbk1 (syst. YNL161w , bit-score=45.5, alignment length=72 aa, e -value=9.7 × 10 −14 ), which is involved in cortical growth [30] , cell morphogenesis and vacuolar organization in yeast (see Supplementary Discussion ) [31] . The contig05937 transcript was weakly homologous to the homeodomain transcriptional repressor Yox1 (syst. YML027w , bit-score=45.2, alignment length=245 aa, e -value=2.6 × 10 −4 ), which in yeast restricts transcription during the cell cycle to the early G1 phase and, when overexpressed, decreases the rate of vegetative growth and delays further progression of the cell cycle, while prolonging the S phase (see Supplementary Discussion ) [32] . The most similar basidiomycete sequence in the uniprot database (B0DSF2, bit-score=192, alignment length=492, e -value=3.0 × 10 −46 ) came from L. bicolor and also contained a homeodomain, which further corroborates the putative regulatory DNA-binding function of contig05937. Pathway analysis Unique among all full-genome-sequenced Hymenoptera, the leaf-cutting ants A. echinatior [33] and A. cephalotes [34] are unable to synthesize arginine because they lack central enzymes in the arginine synthesis pathway. Our fungal pathway analysis showed that the L. gongylophorus transcriptome contained transcripts encoding all enzymes in the urea cycle of the arginine pathway ( Fig. 3a ), but none of these enzyme-coding transcripts were significantly upregulated in gongylidia, except for a few marginally upregulated arginase (Enzyme Commission (EC) 3.5.3.1) transcripts ( Supplementary Table 7 ). We searched the Kyoto Encyclopedia of Genes and Genomes-annotated L. gongylophorus transcriptome data for complete amino acid synthesis pathways with more than one upregulated enzyme in gongylidia. This showed that a single complete set of central enzymes in the phenylalanine and tyrosine synthesis pathway was present in addition to a prephanate dehydratase (EC 4.2.1.51) in the phenylalanine synthesis pathway ( Fig. 3b ). Most transcripts of two central enzymes in this pathway, chorismate mutase (EC 5.4.99.5) and aminotransferase (EC 2.6.1.1), were significantly upregulated in gongylidia ( Fig. 3b and Supplementary Table 8 ). Figure 3: Fungal symbiont genes coding for enzymes involved in the arginine and phenylalanine synthesis pathways. ( a ) The host ant A. echinatior has lost the two enzymes argininosuccinate synthase (EC 6.3.4.5) and argininosuccinate lyase (EC 4.3.2.1) [33] , but the present transcriptome analysis shows that the L. gongylophorus symbiont possesses all the necessary enzymes for arginine synthesis ( Supplementary Table 7 ). Ornithine carbamoyl-transferase (EC 2.1.3.3) was not found among any of the five Hymenopteran insects ( A. cephalotes , Camponotus floridanus , Harpegnathus saltator , Apis mellifera , Nasonia vitripennis ) that were previously analysed [34] , but was also identified in the L. gongylophorus transcriptome. ( b ) Two genes coding for enzymes mediating aromatic amino acids biosynthesis, chorismate mutase (EC 5.4.99.5) and aminotransferase (EC 2.6.1.1), had alleles that were significantly upregulated in the gongylidia ( Supplementary Table 8 ), indicating that the essential amino acids phenylalanine and tyrosine are produced in high amounts in the gongylidia. Full size image To confirm that this upregulation did not just reflect a downregulation of gene expression in the mycelium, we compared the raw read counts of gongylidia and mycelium with the expression of the same genes in the non-gongylidia-producing Leucoagaricus mycelium cultivated by C. longiscapus ( Supplementary Table 9 ). After Bonferroni adjustments for multiple testing, one chorismate mutase transcript (contig06835: χ 2 =7.54, P =0.006, Supplementary Table 9 ) and two aminotransferase transcripts (contig08281: χ 2 =179.0, P< 0.001; contig10399: χ 2 =88.5, P< 0.001, Supplementary Table 9 ) were significantly upregulated in L. gongylophorus gongylidia compared with that in C. longiscapus mycelium. In addition, the transcript contig06652 was significantly upregulated in gongylida compared with that in C. longiscapus mycelium ( χ 2 =101.8, P< 0.001) and also in L. gongylophorus mycelium, so that expression in gongylidia and mycelium was not significantly different ( χ 2 =3.4, P =0.923, Supplementary Table 9 ). Our final analyses focused on chitinase (EC 3.2.1.14) transcripts that play key roles when fungal cell walls grow, either normally or in a modified way in gongylidia and staphylae. Chitinases together with N-acetylglucosaminidase and N-acetylglucosamine kinase are involved in modifying fungal cell walls during hyphal growth and are responsible for chitin recycling and hydrolysis of the N-acetyl- β - D -glucosaminide(1–4)- β -linkages in chitin molecules [35] ( Supplementary Table 10 ). Five of the chitinase transcripts were more than sixfold upregulated in gongylidia compared with that in mycelium (log 2 fold-change=2.65–2.84, Supplementary Table 10 ), whereas two transcripts were more than twofold downregulated ( Supplementary Table 10 ). Most of the remaining chitinase transcripts (53%; 18/34) also showed significant but less than twofold up- or downregulation in gongylidia versus in mycelium ( Supplementary Table 10 ), indicating comprehensive transcriptional modification of the entire chitin synthesis and recycling machinery in gongylidia. The gongylidia of attine ant fungal symbionts have been known since 1893, when Möller [36] first described their basic structure and hypothesized that they were meant to feed the farming ants. Scattered observations of gongylidia in lower-attine fungus gardens suggests that gongylidia-like structures may have evolved several times [37] , but it was only when the fungal cultivar became obligate 20–25 MYA that gongylidia became synamoporphic for all higher-attine (including leaf-cutting) ant fungus gardens. Their functional significance for nutritional provisioning was confirmed more than 30 years ago, and around the same time it was discovered that fungal enzymes are transferred via the ant faecal fluid [13] , [17] . However, the co-evolutionary processes that shaped and maintained these fungal organs have only recently regained focal attention, confirming and expanding the results by Boyd and Martin [17] for a number of fungal enzymes [19] , [20] , [21] . The present study widens this perspective by addressing the fundamental adaptations of gongylidia and the staphylae organs carrying them, and their functional role as storage organs of plant-degrading enzymes and essential amino acids. If gongylidia morphology had differed significantly across gardens maintained by the higher attine genera and species, it would have indicated secondary modification of gongylidia morphology that could have compromised comparisons between lineages that separated ca . 20 MYA, that is, C. longiscapus ant cultivars without gongylidia and the 2–4 MYA L. gongylophorus cultivar [11] . Our finding ( Fig. 1e ) that gongylidia hyphal-tip morphology hardly changed, as this unique cell type evolved ensures that our comparative transcriptomic approach is valid and suitable to address fundamental questions about the specificity of functional gongylidia adaptation. The conserved gongylidia morphology contrasts with the substantial size and number variation in the staphylae that package and distribute the gongylidia across fungus gardens. This is not unlike metazoan organs whose core functional modules represent uniquely conserved evolutionary innovations (for example, neurons, muscle cells and excretory cells), which became elaborated via organic structures that organized them to meet more specific demands as lineages diverged. L. gongylophorus gongylidia have earlier been described as large inflated cells at the tip of growing hyphae that mainly consist of a single, large vacuole [38] . The factors that govern the transition from normal apical hyphal growth to the formation of gongylidia are unknown, although ant pruning behaviours are known to induce staphylae formation in the fungus garden of Atta sexdens [39] . Polarized (apical) growth in filamentous fungi normally responds to external (physical or chemical) and/or internal stimuli that activate and recruit cell-membrane-associated Rho GTPase modules. These transduce the positional signal to the morphogenetic cell machinery, which include the actin cytoskeleton, the polarisome and ARP2/3 complexes, the microtubules and the vesicle trafficking system [40] . Our transcriptomic analyses indicate that gongylidia evolved via condition-dependent modification of gene expression processes that arrest hyphal tip growth, because several differentially expressed transcripts had significant sequence similarity to genes known to be involved in modifying fungal cell metabolism, cytoskeleton regulation, cell wall biogenesis and cell-cycle control ( Fig. 2 , Supplementary Discussion and Supplementary Tables 5 and 6 ). The peculiar cell morphology of L. gongylophorus gongylidia builds up gradually during apical growth and is mainly characterized by the expanding internal cell vacuole [41] . A possible mechanism mediating this process may be a constant influx of proteins, as that would be consistent with the observed shifts in polarity and cell wall biosynthesis (see Supplementary Discussion ) caused by increasing turgor pressure. When grown on agar plates without ants, L. gongylophorus also readily produces gongylidia, but with a lag period because they appear on the surface of the mycelium well behind the expanding growth edge of the mycelium ( Supplementary Fig. 4 ). This suggests that gongylidia formation is induced by depletion of particular nutritional components in the agar, which would be consistent with the stratified occurrence of staphylae mainly in the central section of natural fungus gardens. It is here that fungal garden biomass has probably reached its maximal density and the availability of substrate nutrients starts to become limited for the first time, as the ants inoculated this particular layer of fungus garden with new plant material at the actively growing top of the garden [18] , [20] . The evolutionarily conserved morphology of gongylidia is unlikely to have constrained further co-evolutionary biochemical adaptation, as fundamental partner dependency may lead to genomic reduction of complementary pathways when obligate nutritional interactions last long enough [5] , [42] , [43] . The recently sequenced genomes of A. echinatior and A. cephalotes showed that these two leaf-cutting ants lack two essential genes for arginine biosynthesis that three other genome-sequenced ant species with normal hunter–gatherer life styles have retained [33] , [34] . Both papers hypothesized that the ensuing inability of these ants to synthesize arginine would probably be compensated by metabolic activities of the fungus-garden symbiont. Our present pathway analysis of fungal arginine biosynthesis confirms this hypothesis of nutritional complementarity by showing that L. gongylophorus has the complete set of genes required for arginine biosynthesis ( Fig. 3 and Supplementary Table 7 ). However, none of these transcripts were significantly upregulated in gongylidia relative to mycelium, suggesting that arginine is unlikely to be a limiting essential amino acid in the symbiosis and that other amino acids are in higher demand. This seems particularly probable for phenylalanine and tyrosine, as they belong to the most expensive (ATP-demanding) amino acids to produce [44] . For most immature insects, phenylalanine is an essential amino acid for cuticle production, but not tyrosine, because insect phenylalanine 4-monooxygenase (EC 1.14.16.1) can convert phenylalanine to tyrosine [45] . To avoid growth deficiencies during sclerotization, insect larvae thus need to obtain phenylalanine through their diet, to ensure they can produce tyrosine, dihydroxyphenylalanine (DOPA) and dopamine that are crucial for melanization immune responses and cuticular sclerotization [46] . It is interesting, therefore, that one of the structurally modified and significantly upregulated transcripts in gongylidia was homologous to chorismate mutase ( Supplementary Table 8 ), which belongs to the phenylalanine/tyrosine branch of the aromatic amino acid biosynthesis pathway ( Fig. 3b ) [47] . Analysis of the L. gongylophorus transcriptome further revealed transcripts homologous to the entire phenylalanine/tyrosine pathway and showed that another key enzyme in this pathway, aminotransferase, was upregulated in gongylidia as well ( Fig. 3b and Supplementary Tables 8 and 9 ). Chorismate mutase is a branch-point enzyme between phenylalanine and tyrosine biosynthesis, and is central for the regulation of this pathway in S. cerevisiae , as it is inhibited via a negative feedback loop by tyrosine but not phenylalanine [47] . The upregulation of central enzymes in the phenylalanine biosynthesis pathway indicates that phenylalanine production may be specifically concentrated in gongylidia, consistent with the ant larvae being exclusively fed with gongylidia until they pupate and hatch as adults [48] . Phenylalanine is also transferred to the adult ants as the rectal fluid of the leaf-cutting ant Atta colombica contains 1.09±0.10 μM free phenylalanine per worker [49] . This phenylalanine production is independent of the plant material that the ants offer as fungal substrate, because 3.86 mg free and 7.33 mg protein-bound phenylalanine could be extracted per gram dry weight of L. gongylophorus grown on Potato Dextrose Agar [50] . Genes encoding enzymes for part of the aromatic amino acid biosynthesis pathway have also been discovered among Klebsiella , Enterobacter , Pantoea and Pseudomonas bacteria in A. colombica fungus gardens [51] , suggesting that bacterial symbionts may contribute phenylalanine to the symbiosis as well. Filamentous fungi normally grow by extending their hyphae into the surrounding substrate, ultimately forming a dense hyphal network. When such mycelia grow, amino acids are normally concentrated in vacuoles inside the hyphae from where they are released into the cytoplasm under conditions of nitrogen deficiency [52] . Domesticated fungal cultivars of higher attine (including leaf-cutting) ants grow in a specific stratified manner. The new garden growth in the top section consists mostly of plant substrate with rather few hyphae that are actively colonizing the new plant material. This is followed by productive but saturated fungus garden growth in central garden sections, where hyphae meet their first resource constraints, and ends with depleted garden substrate and old fungal material in the bottom sections that are discarded by the ants [18] . This particular growth form may imply that amino acids concentrated in gongylidia vacuoles may initially have been released when resource constraints started to limit hyphal growth. This would probably have induced the ants to concentrate harvesting in these middle-age central garden sections, where fungal surplus production could no longer be turned into further hyphal growth. This is consistent with the observation that L. gongylophorus does not have a special nutritional composition to encourage unconditional insect mycophagy [12] , as also the lower attine ants whose fungi do not have gongylidia are expected to harvest most prudently when focusing on hyphal tips of resource-limited mycelium. If these inferences are correct, it would suggest that the real innovation of the higher attine symbiont gongylidia consisted in stopping automatic release of amino acids by compartmentalizing enzymes, amino acids and nutrients; hence, the need for more storage compartments could be triggered by ant pruning (further reducing resource availability) [39] and consumption by gongylidia clipping would minimize waste. Recent studies have shed considerable light on the biochemical and molecular details of degradation processes in attine fungus gardens [14] , [18] , [26] , [53] , [54] , emphasizing the importance of fungal carbohydrate-degrading enzymes for rapid and efficient leaf degradation. Gongylidia are important in this process because of the produced and stored enzymes for later ant ingestion and transfer to newly ant-processed plant substrate via faecal fluid [19] . Specifically, the upregulation of a laccase [20] , six pectinases [19] and six proteinases [21] in gongylidia ensures high efficiency of initial leaf degradation [18] . The present transcriptome analysis supports the hypothesis that carbohydrate-active enzymes important for plant material degradation are upregulated in gongylidia and adds the contig03063 GH12 xyloglucanase xeg1 (UniProt accession code U6NF03) to the list of significantly upregulated extracellular gongylidia enzymes ( Supplementary Table 3 ). Expression of this xyloglucanase peaks in the bottom of gardens [55] where many more cellulolytic enzymes are overexpressed [26] , [53] , [55] , but the overexpression in gongylidia suggests that xyloglucanase may also be transferred to the top of fungus gardens via faecal droplets. A previously identified metalloprotease was confirmed to be upregulated in gongylidia [21] , and shown to have a dN/dS ratio >0.5 ( Supplementary Table 6 ) relative to C. longiscapus cultivars without gongylidia whose common ancestor goes at least 25 million years back. This strongly suggests that this enzyme has been modified during coevolution with the fungus-growing ants, but we were unable to verify whether these modifications occurred in relation to the evolution of leaf-cutting ca . 10 MYA or earlier when the gongylidia evolved 20–25 MYA. To our knowledge, only a detoxifying laccase enzyme has been documented to be upregulated also in gongylidia of higher (but non-leaf-cutting) attine ant fungus gardens [20] . However, it would not be surprising if carbohydrate-degrading enzymes in Trachymyrmex and Sericomyrmex fungus gardens would have at least some modified sets of upregulated enzymes compared with L. gongylophorus cultivated by leaf-cutting ants, if these would have specific adaptive functions in the less conspicuous trophic niche of these smaller-colony species. Our present study used molecular techniques to unravel some of the fundamental characteristics of the ‘eat me’ swollen hyphal tips produced by the fungal cultivar of the monophyletic higher attine ants. This innovation 20–25 MYA marked the true domestication of a single lineage of fungal symbiont and allowed it to start co-evolving with the ants because gene flow with free-living relatives became impossible—a development that triggered a massive stepwise increase in ant colony size [9] , division of labour via polymorphic worker castes [7] , chimeric colonies when the ancestor of the leaf-cutting ants switched to multiple queen mating [56] and enhanced prophylaxis via enlarged metapleural glands [57] . As it seems, all this was triggered by the simple beginning of fixing genetic traits that ensured hyphal tips with enlarged vacuoles to become nutrient storage compartments that could be managed by the ants, both for optimal growth and controlled harvest. Once these staphylae organs with gongylidia had evolved, selection for joint symbiotic efficiency could start to elaborate fungal gene expression in these gongylidia to provide spectra of nutrients in proportion to the requirements of each specific attine ant farming symbiosis. Most of these co-evolutionary adaptations remain to be uncovered. Analysis of gongylidia growth characteristics Fungus-growing ant colonies of A. colombica ( n =3), A. cephalotes ( n =3), A . sexdens ( n =3), A. echinatior ( n =3), A. octospinosus ( n =5), A. volcanus ( n =2), Trachymyrmex cornetzi ( n =3), Trachymyrmex zeteki ( n =3), Trachymyrmex opulentus ( n =3), Trissolcus urichi ( n =1), T. sp. 3 ( n =3), T. sp. 10 ( n =3), and Sorbus amabilis ( n =1) were collected in Panama (Gamboa and forests along Pipeline Road), throughout May 2010. Trachymyrmex sp. 3 and T. sp. 10 belong, respectively, to the Trachymyrmex intermedius clade and Sericomyrmex clades in the higher-attine phylogeny [9] and await formal description. Within hours of collection, several staphylae were collected and preserved on microscope slides in a 1% Congo Red, 20% glycerol solution and sealed with nail polish. The diameter of gongylidia was estimated as the average diameter of at least ten individual gongylidia from several staphylae. To measure size and number of staphylae per mm 2 fungus garden area, several small pieces were placed under a stereomicroscope at × 40 magnification after which a 3 × 3 mm square (9 mm 2 ) was randomly placed on these garden fragments ten times to produce replicate counts of the number of staphylae and the mean area that they covered per mm 2 surface area of fungus garden. Non-parametric Kruskal–Wallis tests were used to compare measurements between species using R (R Development Core Team). Excluding species with less than three measured colonies did not change the results of the statistical analysis. RNA extraction and transcriptome sequencing Entire colonies of A. echinatior and C. longiscapus were collected with their fungus gardens in Gamboa, Panama, and transported to the University of Copenhagen, Denmark, where they were maintained at 75% humidity and 25 °C on a diet of bramble leaves, pieces of fruit and dry rice ( A. echinatior ) or oats, catkins and polenta ( C. longiscapus ). Fungal cultivar material was collected from normally growing laboratory colonies of A. echinatior with ~1.5 l of fungus garden. Staphylae (clusters of gongylidia) and mycelium were collected separately with fine flame-sterilized forceps from smaller fragments of fungus garden placed under a microscope ( × 20– × 40 magnification) and immediately placed in 2 ml eppendorf tubes floating in liquid nitrogen. Staphylae are visible on the surface of fungus gardens where they can be collected with minimal adhering mycelium. Extreme care was taken to ensure that no staphylae or individual gongylidia were included in the mycelial fraction. Fungus garden fragments were replaced every 5–10 min, to prevent possible desiccation affecting gene expression in the sampled gongylidia and mycelium. RNA was first extracted separately from ~25 mg (frozen weight) staphylae and mycelium of L. gongylophorus from each of three colonies of A. echinatior ( Ae322 , Ae331 and Ae376 ). The mycelium fraction of the fungus garden from two colonies of C. longiscapus ( jl130511-03 and rmma110512-01 ) was extracted similarly, yielding eight samples in total. C. longiscapus is a lower-attine species that cultivates undifferentiated fungi that do not produce gongylidia, so that only RNA from the mycelial fraction could be extracted ( Fig. 1c ). The fungal tissue was lysed with a FastPrep sample preparation machine (Qbiogene, MP Biomedicals, Santa Ana, California) at 4.5 m s −1 for 45 s in 700 μl RLC lysis buffer (Qiagen, Germany), 7 μl β-mercaptoethanol and glassbeads. The RNA was extracted with an equal volume of phenol/chloroform/isoamyl alcohol (25:24:1), pH 8, followed by an additional extraction with chloroform/isoamyl alcohol (24:1). Final purification of RNA was performed using the RNeasy Plant Mini Kit (Qiagen, Germany, 74903), including an on-column DNase I treatment step as described in the protocol (Qiagen, 79254). The messenger RNA libraries were each tagged and prepared from 2 μg total RNA using TruSeq DNA sample preparation (Illumina, Inc., San Diego, CA) and sequenced as an 8-sample run on a single HiSeq2000 Illumina flowcell yielding 15–20 million single-end 50 bp reads per library by IGA Technology Services S.R.L. (Udine, Italy). In a second round of RNA extractions, ca . 100 mg (frozen weight) of both staphylae and mycelium were collected from colony Ae322 and extracted as described above, but using the RNeasy Midi kit (Qiagen, 75142). The mRNA libraries were prepared from 91.9 μg total staphylae RNA and 109.7 μg total mycelium RNA, respectively, using the Absolutely mRNA Purification Kit (Agilent Technologies—Stratagene, Santa Clara, CA, 400806). Following emulsion PCR amplification, these two libraries were shotgun sequenced on half a plate each using Roche 454 FLX GS Titanium chemistry at the DNA Sequencing Facility, Department of Biology, Lund University, Sweden. Transcriptome assembly and annotation Raw reads were trimmed and filtered to remove low-quality bases, polyA-tails and rRNA. A two-step procedure was used to de-novo assemble all reads (454 and Illumina) from colony Ae322 into a single L. gongylophorus reference transcriptome. First, staphylae and mycelium 454 sequence reads ( Table 1 ) were assembled with MIRA v3.2.1 (ref. 58 ) with standard settings ( job=denovo,est,normal,454 ) in addition to -CO:asir=yes and -CL:ascdc=yes , which treat individual basepair differences as single-nucleotide polymorphisms instead of separate loci and invoke a SKIM routine to reduce the formation of chimeric assemblies by splitting contigs that were linked only by very few reads. Staphylae and mycelium Illumina reads from colony Ae322 ( Table 1 ) were assembled using the Trinity package [59] , with a kmer size of 25 obtained with the Jellyfish counting algorithm. Second, contigs from the MIRA3 and Trinity assemblies with at least 50 bp overlap and 90% identity were assembled using cap3 (ref. 60 ) and final transcripts smaller than 200 bp were discarded. This reduced the total number of transcripts from 45,832 to 23,110, and the reference transcriptome of L. gongylophorus therefore represents individual transcripts with a 90% sequence similarity threshold and thus includes allelic variants of the same locus that are >10% divergent. Functional annotation of the transcriptome assembly was performed by sequence comparison with the UniProtKB database (Release 2012_6, http://www.uniprot.org/ ) using blastx ( e -value<1 e −6) [61] . PFAM domains were assigned by searching the PFAM database [62] with a six-frame protein translation of the assembled contigs. Gene names and Gene Ontology annotations in the UniProt database ( http://www.geneontology.org ) were assigned to assembled contigs in the transcriptome based on the single best hit. KOGs, EC numbers and Kyoto Encyclopedia of Genes and Genomes pathway annotations were assigned using WebMGA [63] . Biological contaminations from microbes co-occurring in the fungus garden were identified by analysing the taxonomic position of the single best UniProt match using Megan, and by blastn ( e -value<1 e −10) searches of assembled transcripts to genomic sequences representing a ca . 7 × coverage draft genome of L. gongylophorus previously published [20] . To evaluate genomic coverage, the assembled transcriptomes were compared with the filtered protein models of available agaric genomes: A. bisporus var. bisporus (H97) v2.0, C. cinerea (BROAD models) and L. bicolor v2.0 using the bidirectional best hits of blastx/tblastn searches ( e -value<1 e −10). Putative repetitive elements were identified by blast searches ( e -value<1 e −10) against a downloaded (July 2012) version of the RepBase database. Profiling tissue-specific gene expression with RNA sequencing Filtered reads from six Illumina libraries (staphylae and mycelium fractions from colonies: Ae322 , Ae331 and Ae376 ) were mapped to the reference transcriptome using bowtie2 (ref. 64 ). For each Illumina read, only the single best mapping position to the assembled transcripts was reported, using gap open and extension penalties of 5 and 3, respectively, and searching up to 100 alternative mapping positions and randomly assigning the mapping position among the best mapping positions for reads that mapped to multiple locations in the transcriptome. The number of reads mapping to each transcript were compiled per sample using mpileup in samtools ver. 0.1.18 (ref. 65 ) and filtered so that only transcripts detected repeatedly (two or more reads mapped in each of the six samples) were used in expression comparisons. All expression data were normalized using a weighted trimmed mean of the log expression ratios (trimmed mean of M -values) to account for compositional bias between RNA libraries as implemented in edgeR [66] . This empirical method adjusts for library size and the potential presence of highly expressed transcripts, leading to underestimation of the remaining read counts. As gongylidia and mycelium samples were ‘paired’ (or ‘nested’) within ant colonies, a linear model with colony as blocking factor was fitted as a negative binomial generalized linear model, with gene-wise dispersion estimated by the Cox-Reid adjusted profile likelihood [67] . Generalized linear model likelihood ratio tests as implemented in edgeR were then used to determine differential expression between gongylidia and mycelium, with the false discovery rate controlled at α =0.05 with the Benjamini–Hochberg method. Only considering transcripts with either Pfam or KOG annotations, a core set of significantly upregulated transcripts was compared with the total set of transcripts with the hypergeometric distribution (that is, sampling without replacement) using the phyper function in R for transcripts annotated with Pfam or KOG, repectively. dN/dS analysis of molecular divergence BLAT ver. 3.0.4 and pslReps [68] was used to uniquely map Illumina reads from the non-gongylidia producing fungus garden of two C. longiscapus colonies to a version of the L. gongylophorus reference transcriptome that only contained Illumina reads. The 454 reads were removed to avoid potentially scoring sequence differences resulting from differences in the error structure of the 454 and Illumina sequencing methods. The consensus sequences of mapped C. longiscapus reads to each transcript were retrieved using samtools ver. 0.1.18. This mapping-based transcript generation was chosen because insufficient read depth of the 50 bp single-end Illumina reads precluded de-novo assembly of a functional C. longiscapus fungus cultivar transcriptome. One-to-one putative orthologous transcript pairs were inferred based on bidirectional best blast ( e -value=1 e −50) hits (bbh). The L. gongylophorus ORFs (beginning with any codon) were retrieved with getorf from the EMBOSS package and aligned in-frame for each L. gongylophorus and C. longiscapus transcript pair. Pairwise non-synonymous and synonymous substitution rates per site (dN/dS) were estimated for each aligned ORF (beginning with any codon) by the Goldman and Yang [69] method using the programme codeml implemented in PAML ver. 4.4b [70] . Only orthologous transcript alignments longer than 300 bp and containing three or more single-nucleotide polymorphisms were included in the analyses. Transcripts were grouped into up-, down- and non-regulated categories based on log 2 fold-change>1,<−1 and between −1 and 1, respectively, and the mean dN/dS ratios compared with Welch’s t -test to control for unequal variances. As an order of magnitude more orthologous transcript pairs were not significantly up- or downregulated, dN/dS ratios were randomly chosen among the non-regulated transcripts using the subset function implemented in R to get equal sample sizes in the two tests. Accession codes: The DNA sequences have been deposited in the European Nucleotide Archive (ENA) under Bioproject accession code PRJEB4168 (ERP003429). The assembled transcriptomes have been deposited in the ENA database under accession codes HAAN01000001 to HAAN01023110 . How to cite this article : De Fine Licht, H. H. et al. Symbiotic adaptations in the fungal cultivar of leaf-cutting ants. Nat. Commun. 5:5675 doi: 10.1038/ncomms6675 (2014).